STAT3 regulated ARF expression suppresses prostate cancer metastasis Prostate cancer (PCa) is the most prevalent cancer in men. Hyperactive STAT3 is thought to be oncogenic in PCa. However, targeting of the IL-6/STAT3 axis in PCa patients has failed to provide therapeutic benefit. Here we show that genetic inactivation of Stat3 or IL-6 signalling in a Pten -deficient PCa mouse model accelerates cancer progression leading to metastasis. Mechanistically, we identify p19 ARF as a direct Stat3 target. Loss of Stat3 signalling disrupts the ARF–Mdm2–p53 tumour suppressor axis bypassing senescence. Strikingly, we also identify STAT3 and CDKN2A mutations in primary human PCa. STAT3 and CDKN2A deletions co-occurred with high frequency in PCa metastases. In accordance, loss of STAT3 and p14 ARF expression in patient tumours correlates with increased risk of disease recurrence and metastatic PCa. Thus, STAT3 and ARF may be prognostic markers to stratify high from low risk PCa patients. Our findings challenge the current discussion on therapeutic benefit or risk of IL-6/STAT3 inhibition. PCa is the second most frequently diagnosed cancer in men with >200,000 new cases reported in the USA annually [1] . Screening for the sensitive yet diagnostically unspecific biomarker prostate-specific antigen (PSA) has led to a substantial rise in the diagnosis of early stage PCa [2] . The failure of current diagnostic tools to reliably distinguish non-aggressive tumours from aggressive ones to predict therapeutic response [3] urgently calls for the identification of better biomarkers to guide treatment. Furthermore, there is need for novel targeted therapies of metastatic PCa based on a better molecular understanding of the disease [4] . The lack of markers to stratify PCa cases into low- and high-risk groups results in overtreatment of 20–42% of patients [5] . STAT3, the major downstream mediator of IL-6 signalling, was shown to be related to advanced tumour growth, by tumour-autonomous mechanisms and by modulating tumour-associated stroma [6] . Although STAT3 activation is observed in ∼ 50% of PCa [7] its functional role in tumorigenesis and metastasis has not been elucidated. Data from the majority of human PCa cancer cell lines support an oncogenic and growth promoting role of IL-6 and STAT3 in vitro [8] . However, metastatic LNCaP cells were growth inhibited in vitro and in vivo in response to IL-6 treatment [8] . Moreover, treatment of patients with an IL-6 blocking antibody did not result in a survival advantage in patients with advanced PCa [9] . Thus, addressing the precise in vivo role of IL-6/STAT3 in PCa is of utmost importance to reassess diagnostic and therapeutic approaches. PTEN is one of the most frequently deleted or mutated tumour suppressors in PCa, with an estimated incidence of 70% in metastatic PCa, causing aberrant activation of the PI3K–AKT–mTOR signalling pathway [10] . Loss of Pten leads to senescence, which is critically regulated by the ARF–p53 pathway [11] . While the tumour suppressor ARF (p14 ARF in humans; p19 ARF in mice) is readily degraded in normal cells, it is stabilized to increase p53 function on loss of Pten. ARF was shown to augment p53 stability by promoting the degradation of Mdm2, a negative regulator of p53. Concomitant inactivation of Pten and p53 leads to bypass of senescence and as a consequence to a malignant PCa phenotype [11] . Previous studies report PTEN–STAT3 signalling crosstalk in malignant glioblastoma [12] , but the detailed molecular mechanisms in cancer progression and metastasis remain unresolved. In this study, we show that loss of IL-6/Stat3 signalling in a Pten -deficient PCa model accelerates cancer progression leading to metastasis. Loss of IL-6/Stat3 signalling in PCa bypasses senescence via disrupting the ARF–Mdm2–p53 tumour suppressor axis. We identify ARF as a novel direct Stat3 target. Notably, loss of STAT3 and p14 ARF expression correlates with increased risk of recurrence in PCa patients. In addition, STAT3 and p14 ARF expression was lost in metastasis compared with the primary tumours. We identified STAT3 and CDKN2A mutations in primary PCa patients. Furthermore, PCa metastases show a high frequency of STAT3 and CDKN2A deletions. We propose STAT3 and ARF as prognostic markers for high versus low risk PCa patient stratification. Co-deletion of Stat3 and Pten triggers PCa To study the role of PTEN and STAT3 in PCa development, we took advantage of mice with conditional loss of Pten in the prostate epithelium ( Pb-Cre4 Pten fl/fl ) hereafter referred to as Pten pc−/− (ref. 13 ). Stat3 protein levels were markedly induced in Pten pc−/− compared with wild-type (WT) prostate epithelium ( Fig. 1a,b ). Pten pc−/− tumours showed strong Akt Ser473 phosphorylation and, unexpectedly, Stat3 Tyr705 and Ser727 phosphorylation suggesting maximal transcriptional activity of Stat3 ( Fig. 1a,b and Supplementary Fig. 1a ). In addition, we observed an increase in IL-6Rα levels in tumour cells and soluble IL-6R serum levels ( Supplementary Fig. 1a–c ) as well as increased Stat3 , IL-6Rα and IL-6 mRNA levels ( Supplementary Fig. 1d ) in Pten pc−/− PCa compared with WT controls. To prove that loss of Stat3 signalling influences PCa formation, we generated mice with concomitant loss of Pten and Stat3 in prostate epithelial cells. Prostate-specific deletion of Pten and Stat3 was confirmed by PCR ( Supplementary Fig. 2a ). Immunohistochemistry (IHC) analysis confirmed loss of pY-Stat3 and Stat3 in Pten pc−/− Stat3 pc−/− tumour cells ( Supplementary Fig. 2b ), while still being present in stromal cells ( Supplementary Fig. 2c ). Surprisingly, and in sharp contrast to the oncogenic role of Stat3 in many cancers [14] , [15] , Pten pc−/− Stat3 pc−/− mice showed accelerated PCa formation with up to sixfold increase in tumour weight compared with Pten pc−/− tumours at different stages of PCa development ( Fig. 1c,d and Supplementary Fig. 2d,e ). Pten pc−/− Stat3 pc−/− tumours showed increased numbers of Ki-67 positive (Ki-67 + ) proliferating cells and reduced numbers of cleaved caspase 3 positive (CC3 + ) apoptotic cells compared with Pten pc−/− prostates ( Fig. 1e,f ). 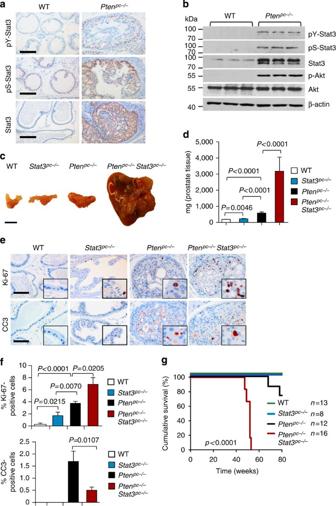Figure 1: Genetic deletion ofStat3andPtentriggers progressive prostate tumorigenesis and lethal disease. (a) Comparison of prostates from WT andPtenpc−/−mice at 19 weeks of age using immunohistochemical (IHC) analysis of pY-Stat3, pS-Stat3 and Stat3. Scale bars, 100 μm. (b) Protein expression analysis of pY-Stat3, pS-Stat3, Stat3, p-Akt, Akt and β-actin with western blots in 19-week-old prostates from WT andPtenpc−/−mice. (c) Gross anatomy of representative prostates isolated at 52 weeks of age from WT,Stat3pc−/−,Ptenpc−/−andPtenpc−/−Stat3pc−/−mice. Scale bars, 10 mm. (d) Prostate weights of 52-week-old WT,Stat3pc−/−,Ptenpc−/−andPtenpc−/−Stat3pc−/−mice (n=24). Mean values are shown; Data were analysed by one-way analysis of variance with Tukey’s multiple comparison test; error bars: s.d. (e) IHC analyses of prostates from 19-week-old WT,Stat3pc−/−,Ptenpc−/−andPtenpc−/−Stat3pc−/−mice stained for Ki-67 and cleaved caspase 3 (CC3). Scale bars, 100 μm; insets: × 600 magnification. (f) Quantification of cells positive for Ki-67 and CC3 using HistoQuest software (n=5). Data were analysed by Student’st-test and are shown as mean±s.d. (g) Kaplan–Meier cumulative survival analysis revealed a significant (P<0.0001; log-rank test) decrease in lifespan ofPtenpc−/−Stat3pc−/−compared withPtenpc−/−mice (n=49); WT andStat3pc−/−mice served as controls. Figure 1: Genetic deletion of Stat3 and Pten triggers progressive prostate tumorigenesis and lethal disease. ( a ) Comparison of prostates from WT and Pten pc−/− mice at 19 weeks of age using immunohistochemical (IHC) analysis of pY-Stat3, pS-Stat3 and Stat3. Scale bars, 100 μm. ( b ) Protein expression analysis of pY-Stat3, pS-Stat3, Stat3, p-Akt, Akt and β-actin with western blots in 19-week-old prostates from WT and Pten pc−/− mice. ( c ) Gross anatomy of representative prostates isolated at 52 weeks of age from WT, Stat3 pc−/− , Pten pc−/− and Pten pc−/− Stat3 pc−/− mice. Scale bars, 10 mm. ( d ) Prostate weights of 52-week-old WT, Stat3 pc−/− , Pten pc−/− and Pten pc−/− Stat3 pc−/− mice ( n =24). Mean values are shown; Data were analysed by one-way analysis of variance with Tukey’s multiple comparison test; error bars: s.d. ( e ) IHC analyses of prostates from 19-week-old WT, Stat3 pc−/− , Pten pc−/− and Pten pc−/− Stat3 pc−/− mice stained for Ki-67 and cleaved caspase 3 (CC3). Scale bars, 100 μm; insets: × 600 magnification. ( f ) Quantification of cells positive for Ki-67 and CC3 using HistoQuest software ( n =5). Data were analysed by Student’s t -test and are shown as mean±s.d. ( g ) Kaplan–Meier cumulative survival analysis revealed a significant ( P <0.0001; log-rank test) decrease in lifespan of Pten pc−/− Stat3 pc−/− compared with Pten pc−/− mice ( n =49); WT and Stat3 pc−/− mice served as controls. Full size image Compared with Pten pc−/− mice [16] , Pten pc−/− Stat3 pc−/− mice displayed a significantly reduced median survival ( Fig. 1g ). Intriguingly, Pten pc−/− Stat3 pc−/− mice developed high-grade (poorly differentiated) PCa with liver and lung metastases ( Fig. 2a ). Histopathological analysis of PCa-bearing animals revealed widespread metastasis in 75% of Pten pc−/− Stat3 pc−/− mice. By contrast, Pten pc−/− mice only showed local invasion into seminal vesicles and never developed distant metastases ( Fig. 2b and Supplementary Table 1 ). Furthermore, loss of Stat3 promoted PCa formation in Pten heterozygous prostate tissue ( Pten pc+/− Stat3 pc−/− ) at 19 weeks of age, whereas Pten pc+/− mice developed only prostatic intraepithelial neoplasia [17] (PIN) ( Supplementary Fig. 3a ). Our data demonstrate that Stat3 suppresses malignant progression of Pten -deficient PCa. We found reduced p53 protein expression in Pten pc+/− Stat3 pc−/− prostates ( Supplementary Fig. 3b ). Pten heterozygosity alone had no effect on p53 expression as demonstrated before [11] . Interestingly, prostate-specific loss of Stat3 ( Stat3 pc−/− ) led to development of PIN lesions in prostates at 19 weeks of age ( Supplementary Fig. 3c ). Analysis of consecutive sections revealed invasive regions and high-grade PIN in Pten pc−/− mice at 19 weeks of age, whereas Pten pc−/− Stat3 pc−/− mice showed early progression to poorly differentiated adenocarcinoma ( Fig. 2c ). At 52 weeks of age Pten pc−/− Stat3 pc−/− tumours had developed into poorly differentiated carcinomas with 86% penetrance compared with Pten pc−/− tumours, which showed only signs of focal invasion and late adenocarcinoma formation ( Fig. 2d ). Notably, Pten pc−/− tumour cells uniformly expressed nuclear Stat3 at 19 weeks of age ( Fig. 2e ), whereas more advanced tumours at 52 weeks of age showed profoundly reduced nuclear Stat3 expression ( Fig. 2e,f ), suggesting that Stat3 expression decreased during PCa progression. 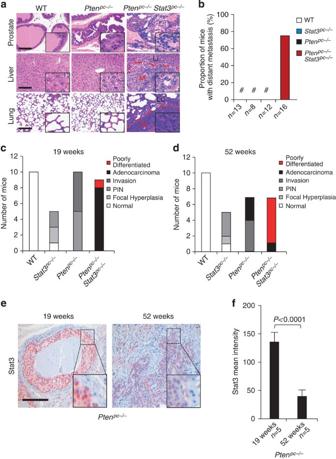Figure 2: Co-deletion ofStat3andPtenenhances prostate cancer transformation and metastatic potential. (a) Histopathological analysis of primary PCa, livers and lungs at 52 weeks of age from WT,Ptenpc−/−andPtenpc−/−Stat3pc−/−mice. The dashed red lines encircle areas of advanced liver or lung metastases (M), which are surrounded by normal liver (Li) or normal lung (Lu), respectively. Scale bars, 100 μm; insets: × 600 magnification. (b) Percentage of mice with sites of distant PCa metastases (n=49). (c) Summary of the histological findings of mouse prostates examined at 19 weeks postpartum (p.p.) from WT,Stat3pc−/−, Ptenpc−/−andPtenpc−/−Stat3pc−/−mice. (d) Summary of the histological findings of mouse prostates examined at 52 weeks p.p. from WT,Stat3pc−/−, Ptenpc−/−andPtenpc−/−Stat3pc−/−mice. Histological grading and classification of mouse prostates was done according to Chenet al.67(e) Stat3 IHC in 19-week- and 52-week-oldPtenpc−/−prostate tumours. Scale bars, 100 μm. (f) Quantification of Stat3 staining in 19-week- and 52-week-oldPtenpc−/−prostate tumours using HistoQuest software,P<0.0001. Data were analysed by Student’st-test and are shown as mean±s.d. (n=5). Figure 2: Co-deletion of Stat3 and Pten enhances prostate cancer transformation and metastatic potential. ( a ) Histopathological analysis of primary PCa, livers and lungs at 52 weeks of age from WT, Pten pc−/− and Pten pc−/− Stat3 pc−/− mice. The dashed red lines encircle areas of advanced liver or lung metastases (M), which are surrounded by normal liver (Li) or normal lung (Lu), respectively. Scale bars, 100 μm; insets: × 600 magnification. ( b ) Percentage of mice with sites of distant PCa metastases ( n =49). ( c ) Summary of the histological findings of mouse prostates examined at 19 weeks postpartum (p.p.) from WT, Stat3 pc−/− , Pten pc−/− and Pten pc−/− Stat3 pc−/− mice. ( d ) Summary of the histological findings of mouse prostates examined at 52 weeks p.p. from WT, Stat3 pc−/− , Pten pc−/− and Pten pc−/− Stat3 pc−/− mice. Histological grading and classification of mouse prostates was done according to Chen et al. [67] ( e ) Stat3 IHC in 19-week- and 52-week-old Pten pc−/− prostate tumours. Scale bars, 100 μm. ( f ) Quantification of Stat3 staining in 19-week- and 52-week-old Pten pc−/− prostate tumours using HistoQuest software, P <0.0001. Data were analysed by Student’s t -test and are shown as mean±s.d. ( n =5). Full size image To further dissect the tumour promoting effects of loss of Stat3, we established primary mouse Pten −/− PCa cells with stable, short hairpin RNA (shRNA) mediated knockdown of Stat3 . Western blot and IHC analyses confirmed efficient Stat3 knockdown in these cells ( Fig. 3a and Supplementary Fig. 4a ). In line with our genetic data, Pten −/− mouse PCa cells with shStat3 knockdown were significantly more invasive in a transwell invasion assay compared with control cells ( Fig. 3b ). We verified the aggressive behaviour of PTEN–STAT3 double deficient tumour cells in an organotypic, physiologically relevant in vitro three-dimensional cancer model [18] . Pten −/− -shStat3 PCa cells displayed a more invasive phenotype compared with control cells in organotypic assays ( Fig. 3c and Supplementary Fig. 4b ). In addition, Pten −/− -shStat3 cells showed increased anchorage-independent cell growth in soft agar compared with Pten −/− PCa cells expressing non-targeting shRNA (control shRNA) ( Fig. 3d ). To corroborate our findings in human cells, combined knockdown of STAT3 and PTEN in human RWPE-1 prostate cells ( Fig. 3e ) increased invasiveness in organotypic assay compared with control and single knockdown cells ( Fig. 3f,g ). Notably, re-expression of STAT3 in human PC3 prostate carcinoma cells, which lack STAT3 expression ( Supplementary Fig. 4c ), led to significantly decreased cell numbers and reduced foci formation ( Fig. 3h and Supplementary Fig. 4d,e ). These data are consistent with a cell-autonomous tumour suppressive role of Stat3 in PCa. 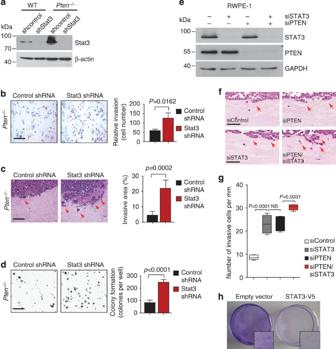Figure 3:Stat3suppresses colony formation and invasion. (a) shRNA-mediated knockdown of Stat3 inPten−/−mouse PCa cells leads to robust decrease of Stat3 levels as demonstrated by western blotting. In all knockdown experiments, scrambled non-target shRNA served as a control (control shRNA/shcontrol). (b) Representative histology of increased matrigel invasion after shRNA-mediated knockdown of Stat3 inPten-deficient (Pten−/−) mouse PCa cells. Quantification of relative invasion is shown (n=3). Scale bars, 100 μm. (c) Organotypic culture assays ofPten−/−mouse PCa cells in the absence of Stat3 showed capacity to invade into the fibroblast containing collagen gel (red arrows). Scale bars, 50 μm. The invasive area/total tumour cell area was quantified (control shRNA,n=4, shStat3n=3). (d) Soft agar colony formation of primaryPten−/−mouse PCa cells with shStat3 and controls was quantified (n=3). Scale bars, 200 μm. Data were analysed by Student’st-test and are shown inc–eas mean±s.d. (e) Efficient STAT3 and PTEN siRNA-mediated knockdown of RWPE-1 cells was demonstrated by western blot. Scrambled non-target siRNA served as a control (control siRNA/siControl) (f) Organotypic culture of RWPE-1 cells in the presence and absence of STAT3 and/or PTEN cultivated in contact with human prostate stromal fibroblasts seeded in collagen I gels after 8 days of culture. Representative H&E stainings are shown, red arrows indicate invasion, scale bars, 100 μm. (n=3). (g) Quantification of invasion of RWPE-1 cells knocked down for PTEN and/or STAT3 using siRNA (number of invasive cells per mm,n=5 sections for each condition). Data were analysed by one-way analysis of variance with Tukey’s multiple comparison test; error bars: s.d. (h) Crystal violet stains of focus formation of STAT3-V5 and empty vector transduced PC3 cells after 4 days of incubation (Supplementary Fig. 4c–e). Figure 3: Stat3 suppresses colony formation and invasion. ( a ) shRNA-mediated knockdown of Stat3 in Pten −/− mouse PCa cells leads to robust decrease of Stat3 levels as demonstrated by western blotting. In all knockdown experiments, scrambled non-target shRNA served as a control (control shRNA/shcontrol). ( b ) Representative histology of increased matrigel invasion after shRNA-mediated knockdown of Stat3 in Pten -deficient ( Pten −/− ) mouse PCa cells. Quantification of relative invasion is shown ( n =3). Scale bars, 100 μm. ( c ) Organotypic culture assays of Pten −/− mouse PCa cells in the absence of Stat3 showed capacity to invade into the fibroblast containing collagen gel (red arrows). Scale bars, 50 μm. The invasive area/total tumour cell area was quantified (control shRNA, n =4, shStat3 n =3). ( d ) Soft agar colony formation of primary Pten −/− mouse PCa cells with shStat3 and controls was quantified ( n =3). Scale bars, 200 μm. Data were analysed by Student’s t -test and are shown in c – e as mean±s.d. ( e ) Efficient STAT3 and PTEN siRNA-mediated knockdown of RWPE-1 cells was demonstrated by western blot. Scrambled non-target siRNA served as a control (control siRNA/siControl) ( f ) Organotypic culture of RWPE-1 cells in the presence and absence of STAT3 and/or PTEN cultivated in contact with human prostate stromal fibroblasts seeded in collagen I gels after 8 days of culture. Representative H&E stainings are shown, red arrows indicate invasion, scale bars, 100 μm. ( n =3). ( g ) Quantification of invasion of RWPE-1 cells knocked down for PTEN and/or STAT3 using siRNA (number of invasive cells per mm, n =5 sections for each condition). Data were analysed by one-way analysis of variance with Tukey’s multiple comparison test; error bars: s.d. ( h ) Crystal violet stains of focus formation of STAT3-V5 and empty vector transduced PC3 cells after 4 days of incubation ( Supplementary Fig. 4c–e ). Full size image Stat3 regulates the ARF–Mdm2–p53pathway Since loss of Pten triggers senescence thereby restricting cancer progression and metastasis [11] , we next tested whether Stat3 exerts a tumour suppressive function by activating senescence-inducing programmes in Pten pc−/− PCa cells [19] at an early stage of PCa development (19 weeks). Senescence is generally characterized by upregulation of p53, cyclin-dependent kinase inhibitor 1 (Cdkn1, p21), promyelocytic leukaemia protein (PML) and elevated senescence-associated-β-galactosidase activity [20] . Of note, Pten pc−/− Stat3 −/− tumours lacked p21 expression, displayed reduced numbers of PML nuclear bodies and decreased SA-β-Gal activity compared with Pten pc−/− tumours ( Fig. 4a,b and Supplementary Fig. 5a,b ), suggesting Stat3 as a novel mediator of senescence in response to loss of Pten. Senescence associated with loss of Pten was shown to be bypassed by deletion of p53 leading to early lethality [11] . We show here that loss of Stat3 and Pten revealed a phenotype strikingly similar to that of p53 and Pten loss [11] . Intriguingly, Stat3 and Pten deletion resulted in downregulation of p53 expression in the prostate epithelium, which was accompanied by the loss of p19 ARF ( Fig. 4a,b ). The p53 expression in the tumour stromal cells remained unchanged ( Supplementary Fig. 5c ). Since p19 ARF is a critical regulator of Mdm2 degradation [21] , our results suggest that the tumour suppressive capacity of Stat3 in senescent tumour cells [22] may rely on the p19 ARF –Mdm2–p53 tumour suppressor axis. 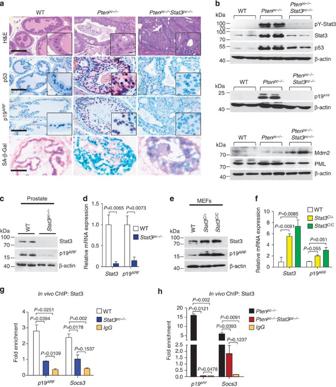Figure 4: Stat3 is a critical regulator of the ARF–Mdm2–p53 tumour suppressor pathway and senescence. (a) Haematoxilin/eosin (H&E) stains show higher grade PCa inPtenpc−/−Stat3pc−/−mice compared withPtenpc−/−mice. Scale bars, 100 μm. IHC analysis of p53, p19ARFand staining for senescence-associated-β-galactosidase activity in prostates from 19-week-old WT,Ptenpc−/−andPtenpc−/−Stat3pc−/−mice. Scale bars, 100 μm; insets: × 600 magnification. (b) Western blot analysis showing pY-Stat3, Stat3, p53, p19ARF, Mdm2 and PML expression levels inPtenpc−/−Stat3pc−/−compared withPtenpc−/−mice. β-actin serves as a loading control. The remaining Stat3 bands inPtenpc−/−Stat3pc−/−prostates are due to Stat3 stromal expression (Supplementary Fig. 2c). (c) Western blot analysis of Stat3 and p19ARFexpression in prostates of 19-week-old WT orStat3pc−/−mice. β-actin serves as a loading control. (d) qRT–PCR analysis ofStat3andp19ARFmRNA expression in prostates of 19-week-old WT orStat3pc−/−mice (n=5 each). Data were analysed by Student’st-test and are shown as mean±s.d. (e) Western blot analysis of Stat3 and p19ARFexpression in WT,Stat3C/+orStat3C/CMEFs. (f) qRT–PCR analysis ofStat3andp19ARFtranscript levels in WT,Stat3C/+andStat3C/CMEFs (n=3 each). Data were analysed by Student’st-test and are shown as mean±s.d. (g)In vivoChIP analysis of Stat3 binding top19ARFandSocs3promoters, respectively, in WT andStat3pc−/−prostate tissue. Stat3 binding to theSocs3(ref.69) promoter, which is a direct Stat3 target served as a positive control. Data were normalized to Cis4200, which served as the negative control70. (h)In vivoChIP analysis of Stat3 binding to thep19ARFandSocs3promoters in PCa. Note the >15-fold enrichment of Stat3 bound to promoter fragments inPtenpc−/−compared withPtenpc−/−Stat3pc−/−tumours. Data ingandhwere analysed by one-way analysis of variance with Tukey’s multiple comparison test and shown as mean±s.d. (Primer pairs are listed inSupplementary Table 2). Figure 4: Stat3 is a critical regulator of the ARF–Mdm2–p53 tumour suppressor pathway and senescence. ( a ) Haematoxilin/eosin (H&E) stains show higher grade PCa in Pten pc−/− Stat3 pc−/− mice compared with Pten pc−/− mice. Scale bars, 100 μm. IHC analysis of p53, p19 ARF and staining for senescence-associated-β-galactosidase activity in prostates from 19-week-old WT, Pten pc−/− and Pten pc−/− Stat3 pc−/− mice. Scale bars, 100 μm; insets: × 600 magnification. ( b ) Western blot analysis showing pY-Stat3, Stat3, p53, p19 ARF , Mdm2 and PML expression levels in Pten pc−/− Stat3 pc−/− compared with Pten pc−/− mice. β-actin serves as a loading control. The remaining Stat3 bands in Pten pc−/− Stat3 pc−/− prostates are due to Stat3 stromal expression ( Supplementary Fig. 2c ). ( c ) Western blot analysis of Stat3 and p19 ARF expression in prostates of 19-week-old WT or Stat3 pc−/− mice. β-actin serves as a loading control. ( d ) qRT–PCR analysis of Stat3 and p19 ARF mRNA expression in prostates of 19-week-old WT or Stat3 pc−/− mice ( n =5 each). Data were analysed by Student’s t -test and are shown as mean±s.d. ( e ) Western blot analysis of Stat3 and p19 ARF expression in WT, Stat3 C/+ or Stat3 C/C MEFs. ( f ) qRT–PCR analysis of Stat3 and p19 ARF transcript levels in WT, Stat3 C/+ and Stat3 C/C MEFs ( n =3 each). Data were analysed by Student’s t -test and are shown as mean±s.d. ( g ) In vivo ChIP analysis of Stat3 binding to p19 ARF and Socs3 promoters, respectively, in WT and Stat3 pc−/− prostate tissue. Stat3 binding to the Socs3 (ref. 69 ) promoter, which is a direct Stat3 target served as a positive control. Data were normalized to Cis4200, which served as the negative control [70] . ( h ) In vivo ChIP analysis of Stat3 binding to the p19 ARF and Socs3 promoters in PCa. Note the >15-fold enrichment of Stat3 bound to promoter fragments in Pten pc−/− compared with Pten pc−/− Stat3 pc−/− tumours. Data in g and h were analysed by one-way analysis of variance with Tukey’s multiple comparison test and shown as mean±s.d. (Primer pairs are listed in Supplementary Table 2 ). Full size image Recently, co-inactivation of p53 and ARF was linked to human triple-negative breast cancer progression through IFNβ–STAT1–ISG15 signalling [23] . Interestingly, ISG15 and Stat3 protein expression levels paralleled each other in the PCa mouse models ( Supplementary Fig. 6a ). This suggests an altered ISGylation system, which could be independent of androgen receptor expression [24] ( Supplementary Fig. 6b ). It is noteworthy, that numerous AR-positive tumour cells were observed in the metastases of the Pten pc−/− Stat3 pc−/− PCa mouse models ( Supplementary Fig. 6c ), underlining the relevance of our model to human PCa [25] . Molecular pathological analysis confirmed AR-positive tumour nodules in five out of five cases of lung metastases consist of 66% AR-positive cells ( Supplementary Fig. 6d ). Mechanistically, Pten was shown to block PI3K-mediated translocation of Mdm2 into the nucleus, where it promotes rapid degradation of p53 (ref. 26 ). In line with the published function of PML to increase p53 stability by sequestering Mdm2 to the nucleolus, disruption of Pten and Stat3 resulted in increased Mdm2 protein levels ( Fig. 4b ). Therefore, loss of Stat3 promotes PCa development by bypassing senescence regulated by the p19 ARF –p53 axis. We therefore hypothesize that Stat3 may act through ARF as an important gatekeeper controlling senescence counteracting metastasis, which we tested further. Immunoblot and IHC analyses revealed a positive correlation between Stat3 and p19 ARF levels. Moreover, loss of Stat3 led to a profound decrease in p19 ARF protein ( Fig. 4a,b ). Transcript levels of the well-established Stat3 target genes Socs3 and c-fos [27] paralleled p19 ARF expression in WT, Pten pc−/− and Pten pc−/− Stat3 pc−/− prostate tissue ( Supplementary Fig. 7a,b ). Stat3 pc−/− prostates displayed a significant decrease in p19 ARF protein and mRNA levels compared with WT controls ( Fig. 4c,d ), suggesting direct regulation of p19 ARF expression by Stat3. We first tested this by analysing p19 ARF expression in passage-matched homozygous Stat3 knockout ( Stat3 KO ) and WT mouse embryonic fibroblasts (MEFs). Both p19 ARF protein and mRNA levels were significantly reduced in the absence of Stat3 ( Supplementary Fig. 7c,d ). Consistently, MEFs expressing one or two hyperactive Stat3 alleles ( Stat3 C/+ and Stat3 C/C ) from the endogenous Stat3 locus [28] displayed upregulation of p19 ARF protein and mRNA ( Fig. 4e,f ). In silico analysis of the p19 ARF promoter [29] predicted two potential Stat3-binding sites ( Supplementary Fig. 7e ). Chromatin immunoprecipitation (ChIP) experiments showed approximately threefold increase in Stat3-binding activity to the proximal p19 ARF promoter region in WT compared with Stat3 pc−/− prostate tissue ( Fig. 4g ). We next wanted to know if Stat3 binding was further elevated in Pten -deficient tumours since Pten loss increased ARF expression. By performing ChIP in Pten pc−/− primary mouse prostate tumours, we demonstrated a 15-fold increase of Stat3 binding to the p19 ARF promoter ( Fig. 4h ), which was abrogated in Pten pc−/− Stat3 pc−/− tumours. These data identify p19 ARF as a novel Stat3 target gene. Loss of IL-6 and Pten leads to cancer and metastasis IL-6 signalling is the major regulator of Stat3 with therapeutic relevance. To address whether Stat3 activation in Pten pc−/− mice depends on IL-6 signalling, we crossed Pten pc−/− mice with IL-6 −/− mice [30] . Co-deletion of IL-6 and Pten triggered early lethality ( Fig. 5a ), progressive high-grade adenocarcinoma formation with increased tumour growth and weight ( Fig. 5b,c ), resulting in disseminated metastases ( Fig. 5d ), for example, in the liver ( Supplementary Fig. 8a ). Loss of IL-6 in Pten heterozygous prostate tissue also resulted in high-grade invasive PCa with metastasis formation at 15 months of age ( Supplementary Fig. 8b ). Like Pten pc−/− Stat3 pc−/− mice, Pten pc−/− IL-6 −/− mice showed markedly enhanced PCa growth ( Supplementary Fig. 8c,d ) at 19 weeks of age, increased Ki-67 + but decreased CC3 + expression levels compared with Pten pc−/− prostates ( Fig. 5e–g ). IHC analysis revealed absence of pY-Stat3 and Stat3 expression in Pten pc−/− IL-6 −/− tumours ( Supplementary Fig. 8e ). 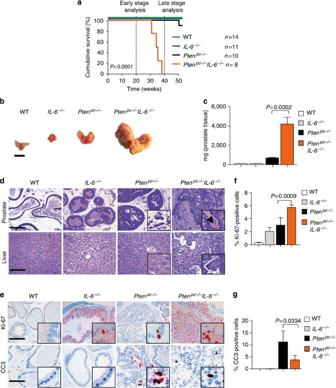Figure 5: Deletion ofIL-6andPtentriggers progressive prostate tumorigenesis and metastatic disease. (a) Kaplan–Meier cumulative survival analysis ofPtenpc−/−IL-6−/−compared withPtenpc−/−mice; WT andIL-6−/−mice served as controls (P<0.0001; log-rank test). (b) Gross anatomy of representative prostates isolated at 38 weeks of age from WT,IL-6−/−,Ptenpc−/−andPtenpc−/−IL-6−/−mice. Scale bars, 10 mm. (c) Prostate weights of 38-week-old WT,IL-6−/−, Ptenpc−/−andPtenpc−/−IL-6−/−mice. Mean values are shown; error bars: s.d. (n=43). (d) Histopathological analysis of haematoxilin/eosin-stained primary PCa and liver at 38 weeks of age from WT,IL-6−/−,Ptenpc−/−andPtenpc−/−IL-6−/−mice. Arrowhead in the inset: area of nerve sheet infiltration. Scale bars, 100 μm. (e) IHC analysis of Ki-67 and CC3 in prostates from 19-week-old WT,IL-6−/−,Ptenpc−/−andPtenpc−/−IL-6−/−mice. Scale bars, 100 μm. (f,g) Bar graphs indicate percentage of cells positive for Ki-67 and CC3 (e). Protein levels quantification was done with HistoQuest software (n=5). Data fromc,fandgwere analysed by Student’st-test and are shown as mean±s.d. Figure 5: Deletion of IL-6 and Pten triggers progressive prostate tumorigenesis and metastatic disease. ( a ) Kaplan–Meier cumulative survival analysis of Pten pc−/− IL-6 −/− compared with Pten pc−/− mice; WT and IL-6 −/− mice served as controls ( P <0.0001; log-rank test). ( b ) Gross anatomy of representative prostates isolated at 38 weeks of age from WT, IL-6 −/− , Pten pc−/− and Pten pc−/− IL-6 −/− mice. Scale bars, 10 mm. ( c ) Prostate weights of 38-week-old WT, IL-6 −/− , Pten pc−/− and Pten pc−/− IL-6 −/− mice. Mean values are shown; error bars: s.d. ( n =43). ( d ) Histopathological analysis of haematoxilin/eosin-stained primary PCa and liver at 38 weeks of age from WT, IL-6 −/− , Pten pc−/− and Pten pc−/− IL-6 −/− mice. Arrowhead in the inset: area of nerve sheet infiltration. Scale bars, 100 μm. ( e ) IHC analysis of Ki-67 and CC3 in prostates from 19-week-old WT, IL-6 −/− , Pten pc−/− and Pten pc−/− IL-6 −/− mice. Scale bars, 100 μm. ( f , g ) Bar graphs indicate percentage of cells positive for Ki-67 and CC3 (e). Protein levels quantification was done with HistoQuest software ( n =5). Data from c , f and g were analysed by Student’s t -test and are shown as mean±s.d. Full size image Intriguingly, in vivo blocking of IL-6/STAT3 signalling by the JAK1/2 inhibitor ruxolitinib in human LNCaP xenografts showed significantly enhanced tumour size and weight ( Fig. 6a,b ). The ruxolitinib-treated xenografts also had markedly increased numbers of Ki-67 + cancer cells accompanied by a decrease in STAT3 and p14 ARF expression ( Fig. 6c ). Moreover, ruxolitinib treatment of LNCaP cells significantly promoted colony formation ( Fig. 6d ). Of note, LNCaP cells lack JAK1 expression and do not respond to interferon signalling [31] . Moreover, STAT3 was shown to be activated in xenografts of LNCaP cells, most likely due to the sole action of JAK2 (refs 32 , 33 ). Ruxolitinib is a dual-specific JAK1/2 kinase inhibitor and therefore, effects of ruxolitinib on the LNCaP xenograft model are likely to be a consequence of JAK2/STAT3 inhibition independent of IFN gamma signalling. 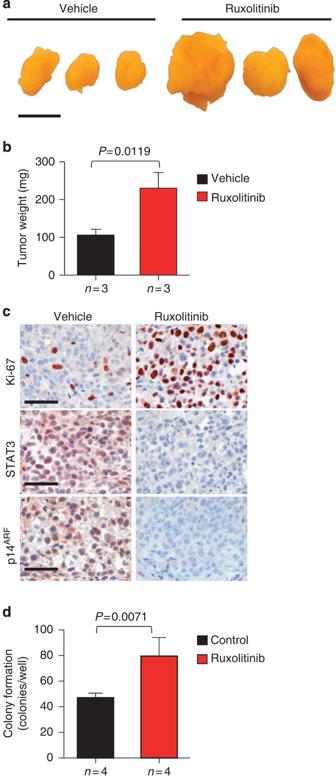Figure 6: JAK1/2 inhibition promotes tumour progression and decreases STAT3 and p14ARFexpression. (a) Gross anatomy of representative LNCaP xenograft tumours treated with ruxolitinib. Mice bearing xenografts were treated with a vehicle or 50 mg kg−1ruxolitinib. Scale bars, 10 mm. (b) Tumour weight of vehicle-treated mice versus ruxolitinib treatment for 22 days of age-matched SCID beige mice. Mean values are shown; error bars: s.d. (n=3). (c) IHC stainings of Ki-67, STAT3 and p14ARFexpression in vehicle versus ruxolitinib-treated xenografted tumours (n=3), scale bar 50 μm. (d) LNCaP cells treated with control (DMSO) or 10 μM ruxolitinib were grown in soft agar for 12 days. Mean values are shown; error bars: s.d. (n=4). Data frombanddwere analysed by Student’st-test. Figure 6: JAK1/2 inhibition promotes tumour progression and decreases STAT3 and p14 ARF expression. ( a ) Gross anatomy of representative LNCaP xenograft tumours treated with ruxolitinib. Mice bearing xenografts were treated with a vehicle or 50 mg kg −1 ruxolitinib. Scale bars, 10 mm. ( b ) Tumour weight of vehicle-treated mice versus ruxolitinib treatment for 22 days of age-matched SCID beige mice. Mean values are shown; error bars: s.d. ( n =3). ( c ) IHC stainings of Ki-67, STAT3 and p14 ARF expression in vehicle versus ruxolitinib-treated xenografted tumours ( n =3), scale bar 50 μm. ( d ) LNCaP cells treated with control (DMSO) or 10 μM ruxolitinib were grown in soft agar for 12 days. Mean values are shown; error bars: s.d. ( n =4). Data from b and d were analysed by Student’s t -test. Full size image Loss of STAT3 and ARF in PCa is associated with metastases The fact that activated STAT3 induces its own transcription [34] led us to measure IL-6 and STAT3 mRNA levels in primary human tumours and to correlate them with clinical outcome. Using the Taylor gene expression profiling data set (GSE21032) [35] , we dichotomized samples based on the z -scores of IL-6 or STAT3 expression. Specifically for IL-6 expression, samples that had z -scores<−2 were defined as low IL-6 and all others ( z -scores>−2) were used as a comparator for prognostic significance. Conversely, samples that had STAT3 z -scores>2 were defined as STAT3 high and all other samples ( z -scores<2) were used as comparators. Time to biochemical recurrence (BCR) was assessed as an indicator of individual prognosis. BCR was defined by an increase to >0.2 ng ml −1 PSA in serum. Of note, patients with low IL-6 expression levels showed a significantly higher risk of BCR compared with patients with high IL-6 expression ( Fig. 7a ). In line, patients with high Stat3 mRNA levels demonstrate good prognosis. This may reflect a higher level of senescence competence compared with patients with lower Stat3 mRNA levels ( Fig. 7b ). 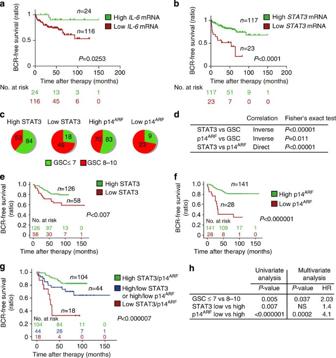Figure 7: Loss of STAT3 and/or p14ARFexpression predicts early BCR in patients with PCa. (a,b) Kaplan–Meier analysis including number at risk of patients stratified into high or lowlL6-andSTAT3mRNA expression predicting biochemical recurrence (BCR) of the Taylor data set35. (c) Distribution of STAT3 and p14ARFprotein expression with low (≤7) or high (8–10) GSC in tumour specimens from men diagnosed with PCa. (d) Fisher’s exact test of data shown incand correlation of STAT3 to p14ARFexpression. (e) Kaplan–Meier analysis of BCR-free survival ratio based on STAT3 protein expression in a panel of 204 PCa patients. (f) Kaplan–Meier analysis of BCR-free survival ratio based on p14ARFprotein expression in a panel of 204 PCa patients. (g) Co-expression analyses of BCR-free survival of STAT3 and p14ARF. (h) Univariate and multivariate analyses of GSC, STAT3 or p14ARFprotein levels. Data froma,b,e,fandgwere analysed by log-rank test. Figure 7: Loss of STAT3 and/or p14 ARF expression predicts early BCR in patients with PCa. ( a , b ) Kaplan–Meier analysis including number at risk of patients stratified into high or low lL6- and STAT3 mRNA expression predicting biochemical recurrence (BCR) of the Taylor data set [35] . ( c ) Distribution of STAT3 and p14 ARF protein expression with low (≤7) or high (8–10) GSC in tumour specimens from men diagnosed with PCa. ( d ) Fisher’s exact test of data shown in c and correlation of STAT3 to p14 ARF expression. ( e ) Kaplan–Meier analysis of BCR-free survival ratio based on STAT3 protein expression in a panel of 204 PCa patients. ( f ) Kaplan–Meier analysis of BCR-free survival ratio based on p14 ARF protein expression in a panel of 204 PCa patients. ( g ) Co-expression analyses of BCR-free survival of STAT3 and p14 ARF . ( h ) Univariate and multivariate analyses of GSC, STAT3 or p14 ARF protein levels. Data from a , b , e , f and g were analysed by log-rank test. Full size image We next tested whether expression of STAT3 and p14 ARF can serve as novel prognostic markers predicting the risk of BCR and metastatic disease progression. STAT3 and p14 ARF levels were independently evaluated by five pathologists in 204 human PCa specimens from patients who underwent radical prostatectomy. Patient samples were categorized into low or high expression groups based on staining intensities and number of positive cells (Methods) using validated antibodies ( Supplementary Fig. 9a,b ). Classification was verified by quantitative histopathological image analysis [36] ( Supplementary Fig. 10a ). Indeed, increased Gleason score (GSC) correlated with low STAT3 or p14 ARF protein expression levels. In addition, we found a strong direct correlation between STAT3 and p14 ARF in accordance with p14 ARF being a direct target of STAT3 ( Fig. 7c,d ). STAT3 expression was significantly decreased in PCa (GCS≤7) compared with PIN areas of 67 matched patient samples ( Supplementary Fig. 10b,c ). Strikingly, both low STAT3 expression ( P <0.007; log-rank test) and low p14 ARF ( P <0.000001; log-rank test) expression were associated with poor outcome ( Fig. 7e,f ). Moreover, combined loss of p14 ARF and STAT3 expression in tumours of PCa patients predicted the worst outcome ( P =0.000007, log-rank test) ( Fig. 7g ). Using multivariate analysis, we identified p14 ARF as a reliable, independent prognostic marker for PCa, which has a twofold higher hazard ratio compared with GSC ( Fig. 7h ). In accordance with the literature [25] , [37] , we found increased AR expression in metastases compared with primary human PCa ( Supplementary Fig. 11a,b ). IHC analysis of matched primary and metastatic human PCa revealed significant loss of PTEN expression in metastatic PCa ( Fig. 8a and Supplementary Fig. 11c ), suggesting an important role of PTEN loss in PCa metastasis. PTEN levels showed no significant correlation with STAT3 or p14 ARF protein expression in a cohort of >200 patients ( Supplementary Fig. 11d,e ). Moreover, we demonstrated that loss of STAT3 and/or p14 ARF is associated with progression to metastatic disease ( Fig. 8b–d ). This is supported by expression data from matched primary and metastatic PCa samples ( Supplementary Fig. 12a–c ), where in all seven cases a significant loss of STAT3 and p14 ARF expression occurred in the metastases. 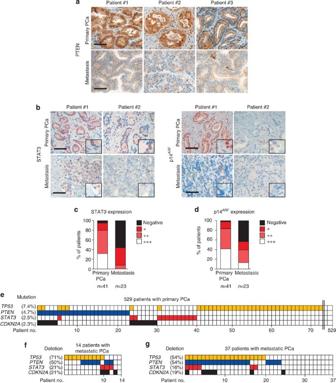Figure 8: Loss of STAT3 and ARF in metastases of PCa patients. (a) Three representative images of PTEN expression determined by IHC analyses in matched patient samples with primary and metastatic PCa (n=5). Scale bars, 100 μm. (b) Representative IHC images of STAT3 and p14ARFexpression from primary (n=41) and metastatic (n=23) PCa samples. Scale bars, 100 μm. (c,d) STAT3 and p14ARFstaining intensity ranging from undetectable (Negative) to maximal expression levels (+++) in cohorts of primary and metastatic PCa. (e) Graphical representation ofTP53,PTEN,STAT3andCDKN2Amutations in 529 patients with primary PCa71. (f) Graphical representation ofTP53,PTEN,STAT3,CDKN2Adeletions in 14 metastatic PCa55. Data were processed by Affymetrix Genome-Wide Human SNP Array 6.0. (g) Graphic representation of gene deletion analysis ofTP53,PTEN,STAT3andCDKN2Ain an independent data set of 37 metastatic PCa samples35. Figure 8: Loss of STAT3 and ARF in metastases of PCa patients. ( a ) Three representative images of PTEN expression determined by IHC analyses in matched patient samples with primary and metastatic PCa ( n =5). Scale bars, 100 μm. ( b ) Representative IHC images of STAT3 and p14 ARF expression from primary ( n =41) and metastatic ( n =23) PCa samples. Scale bars, 100 μm. ( c , d ) STAT3 and p14 ARF staining intensity ranging from undetectable (Negative) to maximal expression levels (+++) in cohorts of primary and metastatic PCa. ( e ) Graphical representation of TP53 , PTEN , STAT3 and CDKN2A mutations in 529 patients with primary PCa 71 . ( f ) Graphical representation of TP53 , PTEN , STAT3 , CDKN2A deletions in 14 metastatic PCa [55] . Data were processed by Affymetrix Genome-Wide Human SNP Array 6.0. ( g ) Graphic representation of gene deletion analysis of TP53 , PTEN , STAT3 and CDKN2A in an independent data set of 37 metastatic PCa samples [35] . Full size image Current data suggest that PCa harbour common genomic and epigenomic alterations [38] , [39] . We analysed large-scale human cancer data sets (International Cancer Genome Consortium (ICGC) and COSMIC databases) and the GEO methylation database [40] . Surprisingly, we found mutations of STAT3 (2.5%) and CDKN2A (2.3%) in a cohort of 529 patients with primary PCa ( Fig. 8e ). We found five missense-, one nonsense- and several conservative STAT3 mutations in primary PCa patients ( Supplementary Fig. 13a ). STAT3 and/or CDKN2A were frequently deleted in metastatic PCa ( Fig. 8f and Supplementary Fig. 13b ), which have been confirmed in an independent data set [35] ( Fig. 8g ). Notably, in 66% of STAT3 deletions, PTEN was co-deleted in both metastases data sets investigated ( Fig. 8f,g ). However, we neither detected human IL-6 mutations nor methylation of STAT3 and CDKN2A loci in primary and metastatic PCa ( Supplementary Figs 13c,d and Supplementary Figs 14a,b ). Due to the lack of prognostic markers for risk stratification, many PCa patients suffer from overtreatment and a severely reduced quality-of-life. Understanding the molecular genetics underlying PCa and the identification of genetic and/or biochemical markers predicting clinical outcome is therefore of high priority. Our data reveal robust upregulation of the IL-6/Stat3 signalling axis in a PCa mouse model as well as in patient specimens. Loss of Stat3 or IL-6 accelerates the progression to metastatic PCa; this stands in sharp contrast to the proposed oncogenic function of IL-6/Stat3 signalling in PCa [33] , [41] , [42] . Moreover, there are contradictory studies on the role of senescence in tumorigenesis [42] , [43] , [44] . Whether these different findings are due to the use of distinct mouse models, strains and species remains to be addressed. Here we combine an array of experimental approaches including in vivo models, mechanistic data with comprehensive human pathological, molecular and genetic data to underscore the tumour suppressive role of STAT3 (ref. 45 ). Thereby we identify STAT3 and its transcriptional target ARF as novel powerful prognostic markers for PCa patients. In PCa and several other cancers, elevated serum IL-6 levels correlate with a poor prognostic outcome for patients [46] . This sparked the development of IL-6 inhibitors to abrogate hyperactive IL-6/STAT3 signalling. However, blocking IL-6/STAT3 signalling was ineffective in patients with advanced PCa [9] , [47] , challenging this oncogenic concept. We show that loss of Stat3 accelerates malignant progression of prostate tumours through abrogation of p19 ARF expression, which we identified as a novel direct Stat3 target gene. Several reports have demonstrated that loss of Pten leads to increased senescence associated with p53 stabilization triggered by p19 ARF (refs 11 , 48 ). Inactivation of Stat3 and Pten revealed striking similarities to the malignant phenotype observed after deletion of Pten and p53 (ref. 11 ). Our model implicates high Stat3 and/or IL-6 levels in senescence-competent PCa and therefore does not contradict the general observation of high IL-6 and/or Stat3 expression in many cancers. We show that impaired p19 ARF expression in Stat3- deficient PCa is accompanied by loss of senescence. In line with our data, concomitant loss of Pten and p19 ARF in MEFs resulted in bypass of senescence, induction of hyperproliferation and oncogenic transformation [11] . Accordingly, overexpression of p19 ARF leads to p53-dependent cell growth arrest and induces senescence [49] . However, systemic p19 ARF deficiency in Pten pc−/− mice did not accelerate PCa or enhance p53 accumulation [50] , which might be explained by inflammatory cytokines and/or growth factors produced by the multiple tumours developing in other organs [51] . Here we identified an unpredicted tumour suppressor role for Stat3 signalling in PCa by its ability to control the tumour suppressor ARF–Mdm2–p53 pathway in a context-dependent manner. Therefore, we propose the STAT3–ARF axis as a previously unknown safeguard mechanism against malignant progression in PCa. Importantly we also demonstrate that loss or inhibition of STAT3–ARF signalling enables tumour progression and metastasis formation. This is reflected in patients with PCa, since loss of STAT3 and/or p14 ARF expression significantly correlates with poor prognosis in large independent data sets. Therefore, our study identifies STAT3 and ARF as potential novel prognostic markers predicting BCR-free survival. The importance of the STAT3–ARF axis is corroborated by the presence of STAT3 mutations in primary PCa and frequent deletions of STAT3 and ARF in metastatic PCa. The significant loss of STAT3 and p14 ARF expression from matched primary and metastatic PCa samples underlines the relevance of our findings. Interestingly, loss of PTEN expression in primary human PCa did not correlate with overall survival [52] and could not predict PCa-specific death [53] . Moreover, heterozygous PTEN deletions far outnumber homozygous deletions in primary human PCa [54] and we show here that PTEN is mutated or lost only in a small subset (4.7%) of a large cohort of patients with primary PCa. However, PTEN is lost in >50% of human PCa metastases [55] , [35] , suggesting an important role for PTEN in this process. Finally, we show in our study that STAT3 is co-deleted with PTEN in 66% of human PCa metastases in two independent data sets. Since PTEN is mutated or lost in only a minor fraction of primary PCa, other aberrations must occur (oncogene induction or loss of tumour suppressor function) to activate STAT3 and ARF to induce senescence in human cancers. Indeed, several studies indicate that different aberrations can lead to induction of senescence in human cancers [48] , [56] . Many human PCa cases are diagnosed with low GSCs, which are of clinical low risk. Only a minority of these tumours will progress to aggressive lethal PCa. We show that ARF is an independent prognostic marker with a twofold higher hazard ratio compared with GSC ( Fig. 7h ). This will enable significantly improved stratification of low risk PCa patients into active surveillance, avoiding severe side effects such as incontinence and/or impotence. Together with a previously defined four-gene signature of aggressive tumours, including PTEN , SMAD4 , CCND1 and SPP1 (ref. 16 ), determination of STAT3 and ARF expression could significantly improve the selection of patients with high risk PCa for personalized anti-cancer treatment. We have uncovered a paradigm shift in understanding the key function of STAT3 in tumorigenicity and metastatic progression in PCa. Therefore, our results call for cautious use of anti-IL-6-STAT3 signalling blockers in the treatment of PCa as this may turn low-grade tumours into highly malignant cancers by loss of senescence controlled by the STAT3–ARF axis. As IL-6/STAT3 signalling blockers are successful in the treatment of chronic inflammatory or autoimmune diseases, their influence on PCa development needs to be carefully evaluated in future studies. Reactivating the IL-6/STAT3/ARF-dependent senescence pathway [57] might be a promising strategy for PCa therapy via downregulation of Mdm2 (ref. 58 ) or p53 induction [59] . Alternatively, triggering ARF–p53-independent cellular senescence by a small molecule inhibitor [60] , could be beneficial for PCa patients in whom other therapies have failed. Generation of transgenic mice Pten loxP/loxP mice crossed with male PB-Cre4 transgenic mice were generated as described previously [13] , [61] . To generate prostate-specific deletion of Pten and IL-6 , we took advantage of IL-6 −/− mice [30] . In a similar strategy, mice carrying Stat3 loxP/loxP [62] were maintained and crossed with PB-Cre4 Pten loxP/loxP transgenic mice. All mice were maintained on a C57BL/6 and Sv/129 mixed genetic background. Animal experiments were reviewed and approved by the Austrian ministry authorities and conducted according to relevant regulatory standards (BMWF-66.009/0281-I/3b/2012). Immunohistochemistry and histological analysis Immunohistochemistry and haematoxilin/eosin staining was performed with formalin-fixed paraffin-embedded (FFPE) tissue using standard protocols using consecutive sections. The following antibodies were used for immunohistochemistry: pY-Stat3 (1:80 dilution; Cell Signaling, #9145), pS-Stat3 (1:80; Cell Signaling, #9134), Stat3 (1:200 dilution; SCBT, sc-7179), p-Akt (1:80 dilution; Cell Signaling, #4060), Akt (1:100 dilution; Cell Signaling, #4691), p53 (1:50 dilution; Calbiochem, pAb421 ), p19 ARF (1:200 dilution; Abcam, ab-80), p14 ARF (1:100 dilution; SCBT, sc-8340), p21 (1:100 dilution; SCBT, sc-397), PML (1:100 dilution; SCBT, sc-966), Ki-67 (1:1,000 dilution; Novocastra; NCL-KI-67-P) and Cleaved Caspase 3 (1:200 dilution; Cell Signaling, #9661) and ISG15 (1:30; Abcam, 131119), AR (1:300; SCBT, sc-816). Staining for SA-ß-Gal activity was performed according to the manufacturer’s protocol (Cell Signaling, #9860). We used PTEN [63] and AR (1:250; DAKO, AR441) [64] antibodies validated for FFPE IHC. The STAT3 antibody was validated using SW620 colon cancer xenografts with shRNA-mediated knockdown ( Supplementary Fig. 9b ). The specificity of p14 ARF antibody was validated using the human melanoma cell lines [65] VM-28 (WT for p14 ARF ) and VM-7 (deletion at the p14 ARF locus). All images were taken with a Zeiss AxioImager Z1, and quantification was performed with HistoQuest (TissueGnostics GmbH, Vienna, Austria, www.tissuegnostics.com ) as described in detail in (ref. 36 ). In brief, haematoxylin staining was used for cell identification. The range of intensities of the master marker (haematoxylin) and the immunohistochemical stainings were set by autodetection of the software. All images were analysed with the identical settings after adjustments. The results are visualized in dot plot scattergrams and/or histograms. Cut-offs (to differentiate between positive and negative cells) and gates (to accentuate between cell populations) were set in the dot blots. For statistical analysis, the raw data were imported into GraphPad Prism 6 (GraphPad Software), analysed for significance and processed for data output. All images were taken with the same exposure time, signal amplification and objectives. Western blot analysis For protein expression analysis by western blot, frozen tissue samples and cell lysates were prepared as described [16] . Blots were blocked with 5% BSA or 5% non-fat dry milk in 1 × TBS/0.1% Tween-20 for 1 h and incubated with the primary antibody overnight at 4 °C. Primary antibodies were reactive to pY-Stat3 (1:500 dilution), pS-Stat3 (1:1,000 dilution), Stat3 (1:1,000 dilution; Cell Signaling, #9132), p19 ARF (1:1,000 dilution), p53 (1:1,000 dilution; Cell Signaling, #2524), p21 (1:500 dilution), β-actin (1:5,000 dilution; Sigma-Aldrich, A5316), p-Akt (1:1,000 dilution), Akt (1:2,000 dilution ), AR (1:1,000 dilution), GAPDH (1:5,000 dilution; Cell Signaling, #2118), Pan-Cytokeratin (1,000 dilution; Abcam, Ab6401), Mdm2 (1:500 dilution; Millipore, 04-1530), PML (1:500 dilution; Millipore, MAB3738) and GAPDH (1:25,000; Trevigen, 2275-PC-100). Supplementary Figures 15–19 show uncropped immunoblots. RNA and qRT–PCR Total RNA was isolated using Trizol (Invitrogen) according to the manufacturer’s instructions. For quantitative reverse transcription PCR (qRT–PCR) analysis, 1 μg of total RNA was reverse transcribed to cDNA using the Transcriptor First-Strand cDNA Synthesis kit (Fermentas). qRT–PCR was performed in triplicate with aa MxPro3000 and SYBR GreenERqPCR mix (Invitrogen). Real-time monitoring of PCR amplification was performed using the LightCycler 480 detection system (Roche). The relative amount of specific mRNA was normalized to β-actin in each sample. Primer pairs are listed in Supplementary Table 3 . Cell culture Primary WT and Stat3 -null MEF were isolated by trypsin treatment of individual littermate E13.5 embryos from a cross of Stat3 +/− heterozygous mice. Stat3 +/− mice were generated from conditional Stat3 +/fl mice [66] by deletion of the conditional allele in vivo using Mox2-Cre . Cells were amplified and used in experiments starting at passage 2. Stat3 −/− MEFs were grown in DMEM supplemented with 10% FBS, 2 mM L-Glutamine, 0.1 mM NEAA, 20 mM HEPES and pen/strep using standard techniques. Stat3 C/+ and Stat3 C/C MEFs were generously provided by Valeria Poli [28] . For in vitro cultures LNCaP, RWPE-1 and PC3 were cultured under standard conditions. Generation of primary mouse prostate cell lines Dissected prostate tissue from WT and Pten pc−/− mice at 19 weeks of age was cut into pieces of 0.2 mm, plated in tissue culture dishes coated with type I collagen (BD Pharmingen) and supplied with a minimal amount of epithelial growth medium containing 1% FBS serum. After 24 and 48 h, more medium was added. After an additional 24–72 h, cells began to grow out from the prostate tissue. Clean epithelial cell lines were obtained by removing the unwanted cell type with a cell scraper or pipette tip. Cells were passaged using Accutase (PAA, L11-00). For the generation of cell lines, cells were passaged until they survived crisis and only cells with typical epithelial morphology were maintained. WT and Pten pc−/− prostate cell lines were established and maintained in DMEM/F12 (Invitrogen, 3133095) plus 10% foetal bovine serum (PAA, A15-101), 25 mg ml −1 bovine pituitary extract (Invitrogen, 13028014), 5 mg ml −1 EGF (Peprotech, 315-09), insulin/transferrin/selenite (Invitrogen, 41400-045), pen/strep (PAA, 30-002-CI), cholera toxin (Sigma-Aldrich, C8052-5MG) and ciprofloxacin (Sigma-Aldrich, 17580-5G). Prostate tumour epithelial cell lines expressed the epithelial marker Pan-Cytokeratin detected by immunofluorescence and western blot analysis. Pten deletion was confirmed by PCR and western blot analysis. Human tissue microarray The human tissue arrays representing a panel of 204 patient samples were obtained from the Institute of Pathology, Tuebingen, Germany and from the Clinical Institute of Pathology (CIP) of the Medical University of Vienna (MUW), Vienna, Austria. The cohort contains tumour material from PCa patients who consecutively underwent radical prostatectomy at the University Hospital of Tuebingen or the University Hospital of the MUW. Each PCa specimen was represented by two cores on tissue microarrays (TMA). From the CIP of the MUW, we furthermore obtained 41 PCa and 23 metastasis FFPE patient samples. In addition, we include FFPE material from 67 matched patient samples with PIN and PCa (GSC≤7), as well as 7 matched patient samples with primary PCa and PCa metastases, all from the CIP, MUW. The FFPE tissue blocks were sectioned as 3-μm-thick sections mounted on slides and stained with haematoxylin and eosin. Subsequently, the area of cancer was marked by a pathologist (S.P.). Cores, each of up to 0.6 mm in diameter, were taken from the corresponding donor block and placed into a TMA recipient block using a semiautomatic tissue arrayer (Beecher Instruments). Tissue sections (3-μm thick) were placed onto superfrost slides. IBM SPSS Statistics 20 (IBM) was used for statistical analysis. For determination of time to BCR, which is defined by an increase to >0.2 ng ml −1 PSA in serum, a log-rank (Mantel–Cox) test was used to test significance. The hazard ratio and its confidence interval were calculated using the Mantel–Haenszel method. All the human samples for TMA and their use in this study were approved by the Research Ethics Committee of the Medical University Vienna, Austria (1753/2014) and by the Research Ethics Committee for Germany (395/2008BO1) (Bonn, Germany). Statistical analyses Data were analysed using GraphPad Prism 6 software. For comparing two groups unpaired Students t -test and for comparing more than two groups Tukeýs post hoc test was used. Fisher’s exact test was employed when differences in distributions within groups were monitored. For Kaplan–Meier analysis and log-rank statistical evaluation of time to BCR, as well as evaluation of prognostic power in univariate and multivariate analysis, we used the IBM SPSS version 22 programme. To analyse Affymetrix SNP Chip 6.0 primary data, we used the AGCCytoScan Software together with the Chromosome Analysis Suite 3.0 (both Affymetrix), and deletions >200 kb were considered significant. For analysis of mutations in primary PCa, we used the ICGC ( www.icgc.org ). ELISA For the detection of soluble sIL-6R in sera of mice, the samples were diluted 1:15 in 1% BSA–PBS. The ELISA was performed as described [67] . In brief, microtiter plates (Greiner Microlon) were coated with anti-murine IL-6-R pAB AF1830 (0.8 μg ml −1 ; R&D Systems) in PBS. After blocking, 100 μl aliquots of cell lysates or culture supernatants were added. IL-6R bound to the plate was detected by biotinylated goat anti-mouse IL-6-R pAB BAF1830 (working concentration, 0.2 μg ml −1 ; R&D Systems) followed by streptavidin–horseradish peroxidase (R&D Systems). The enzymatic reaction was performed with soluble peroxidase substrate (BM blue POD from Roche) at 37 °C and the absorbance was read at 450 nm on a SLT Rainbow plate reader (Tecan). For the detection of murine IL-6 in sera of mice, the samples were diluted 1:3 with 1% BSA–PBS. How to cite this article: Pencik, J. et al. STAT3 regulated ARF expression suppresses prostate cancer metastasis. Nat. Commun. 6:7736 doi: 10.1038/ncomms8736 (2015).